Accumulating the hydride state in the catalytic cycle of [FeFe]-hydrogenases H 2 turnover at the [FeFe]-hydrogenase cofactor (H-cluster) is assumed to follow a reversible heterolytic mechanism, first yielding a proton and a hydrido-species which again is double-oxidized to release another proton. Three of the four presumed catalytic intermediates (H ox , H red /H red and H sred ) were characterized, using various spectroscopic techniques. However, in catalytically active enzyme, the state containing the hydrido-species, which is eponymous for the proposed heterolytic mechanism, has yet only been speculated about. We use different strategies to trap and spectroscopically characterize this transient hydride state (H hyd ) for three wild-type [FeFe]-hydrogenases. Applying a novel set-up for real-time attenuated total-reflection Fourier-transform infrared spectroscopy, we monitor compositional changes in the state-specific infrared signatures of [FeFe]-hydrogenases, varying buffer pH and gas composition. We selectively enrich the equilibrium concentration of H hyd , applying Le Chatelier’s principle by simultaneously increasing substrate and product concentrations (H 2 /H + ). Site-directed manipulation, targeting either the proton-transfer pathway or the adt ligand, significantly enhances H hyd accumulation independent of pH. Hydrogen (H 2 ) turnover in [FeFe]-hydrogenases is proposed to occur at the distal iron site (Fe d ) of the [2Fe2S] moiety (2Fe H ), which is part of the H-cluster [1] . The distal iron ion exchanges protons with a conserved proton-transfer pathway (PTP) [2] , [3] via an azadithiolate ligand (adt) that bridges both iron sites ( Fig. 1 ) [4] , [5] . Different redox states of the H-cluster can be distinguished by the unique infrared vibrational signatures of the two CN − and three CO ligands at the 2Fe H moiety. To tailor [FeFe]-hydrogenases for specific applications or translate their catalytic principle into productive and durable synthetic mimics, detailed knowledge of the succession of turnover steps occurring at the H-cluster is required. The binuclear metal cofactors of [FeFe]- and [NiFe]-hydrogenases have been suggested to oxidize H 2 by enhancing the acidity of H 2 in the presence of a base, thus facilitating its heterolytic cleavage into a proton (H + ) and hydride (H − ) as a first intermediate step ( Fig. 1 ) [6] , [7] , [8] , [9] . 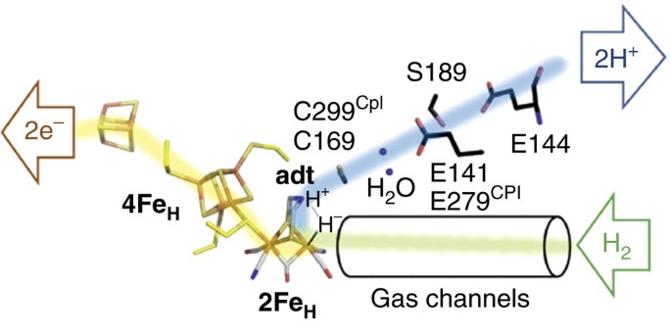Figure 1: Substrate/product transfer and heterolytic H2splitting in [FeFe]-hydrogenases. The electron-transfer path is shown in yellow, the PTP is depicted in blue. H2is released from, or reaches the 2FeHcluster through hydrophobic gas channels (green). At the catalytically pivotal 2FeHsite, the presumptive first step in the catalysis of H2oxidation (H2heterolysis) is depicted, resulting in the unequal intermediates H+, binding at the adt-bridge (Lewis base) and H−, binding at Fed(Lewis acid). Figure 1: Substrate/product transfer and heterolytic H 2 splitting in [FeFe]-hydrogenases. The electron-transfer path is shown in yellow, the PTP is depicted in blue. H 2 is released from, or reaches the 2Fe H cluster through hydrophobic gas channels (green). At the catalytically pivotal 2Fe H site, the presumptive first step in the catalysis of H 2 oxidation (H 2 heterolysis) is depicted, resulting in the unequal intermediates H + , binding at the adt-bridge (Lewis base) and H − , binding at Fe d (Lewis acid). Full size image For [NiFe]-hydrogenases, electron paramagnetic resonance spectroscopy showed that a bridging metal hydride was present in the paramagnetic Ni-C state [6] , [7] , while an ultra-high 0.89 Å resolution X-ray crystallography structure enabled the assignment of both, the proton and bridging hydride, in the first state following H 2 -binding (Ni-R) [8] . For algal-type [FeFe]-hydrogenases, a comparative density functional theory (DFT)/X-ray absorption spectroscopy analysis indicated a bridging hydride (μ-H − ) in the double-reduced H sred state [10] , albeit the importance of a μ-H − state for fast catalytic turnover has been questioned. In fact, the terminal hydride (t-H − ) is thermodynamically less stable and more reactive compared to μ-H − and would match the high turnover kinetics of [FeFe]-hydrogenases far better [11] , [12] , [13] , [14] . According to the current working model for the catalytic mechanism of [FeFe]-hydrogenases [1] , binding of H 2 to the oxidized active ready state (H ox ) results in the heterolytic cleavage of H 2 , with H hyd as the first intermediate. On deprotonation, H hyd is converted into the rather stable H sred state before two successive oxidation steps recycle H ox . A direct conversion of H hyd into H red has been proposed as well [15] . However, a terminal hydride has not been assigned to any of the known redox states [10] , nor has another catalytic wild-type state with the postulated t-H − been reported. This implies that the kinetically relevant hydride state is a transient one and difficult to trap under steady-state conditions. Owing to the rules governing steady-state kinetics, which favour thermodynamically stable intermediates in catalysis, the direct characterization of transient states relies on the utilization of time-resolved approaches with stopped-flow or single-turnover set-ups [16] . We take a different approach, exploiting the properties of steady-state kinetics and using Le Chatelier’s principle to selectively enrich the transient t-H − state in three different [FeFe]-hydrogenases: HydA1; DdH; and CpI, which cover the complete range of increasingly complex structured monomeric hydrogenase subtypes (M1–M3) [17] , [18] , [19] , [20] . In our experimental set-up, attenuated total reflection (ATR) Fourier-transform infrared (FTIR) spectroscopy is used to follow the population of different catalytic states. Compositional changes are monitored in the state-specific infrared signatures as a function of buffer/gas composition. 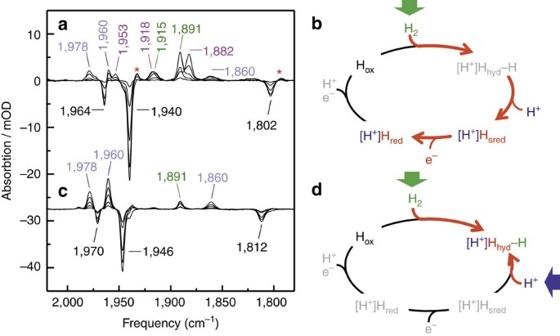Figure 2: Population of Hhydin HydA1 by simultaneously increasing H2and H+pressure. (a) ATR FTIR difference spectrum (N2/pH8→H2/pH8), depicting the accumulation of the reduced states (Hred/Hredand Hsred) in the catalytic cycle of HydA1 under H2at pH 8. (c) ATR FTIR difference spectrum (N2/pH8→H2/pH4) depicting the accumulation of Hhydin the catalytic cycle of HydA1 under H2at pH 4. Catalytic cycles (b,d) beside the corresponding spectra illustrate the shift in steady-state equilibrium depending on applied substrate and product pressures in the working model of the catalytic cycle, which comprises the already-characterized states Hox, Hred/Hredand Hsred, and the missing H2-activated state (Hhyd). Peak labels for Hoxare presented in black, for Hhydin blue, for Hredin green and for Hsredin magenta (red asterisks: Hred). For the complete state-specific CN−-/CO-vibrational spectra of HydA1 observed during sample analysis, seeSupplementary Table 1. At pH 4, the vibrational signals of Hoxwere slightly shifted to higher frequencies (for more information seeSupplementary Table 1, Hox-blue). Accumulation of H hyd in wild-type [FeFe]-hydrogenases Figure 2a depicts FTIR difference spectra of HydA1 film at pH 8 recorded while changing the atmosphere from N 2 to H 2 (for details about the experimental setup see Supplementary Fig. 1). Negative bands mainly comprised the frequency pattern of H ox (1,964/1,940/1,802 cm −1 ). Positive bands included marker frequencies 1,915/1,891 cm −1 (H red ) and 1,953/1,918/1,882 cm −1 (H sred ), corresponding to earlier measurements with H 2 -purged HydA1 carried out in transmission FTIR systems [21] . On steady-state supply of substrate (that is, H 2 ), the enzyme accumulates the apparently rather stable reduced intermediates H red and H sred . However, bands at 1,978/1,960/1,860 cm −1 could be identified as minor contributions, indicating the presence of another state, which resembles the band pattern of H trans in DdH (H trans -like state) [22] and was previously observed as a weak fraction of a complex band pattern in a sodium dithionite (NaDT)-treated HydA1 sample [23] . According to our working model, deprotonation should lead from the presupposed H hyd to the reduced states ( Fig. 2b ), and a plausible way to selectively enrich H hyd would be a simultaneous increase in substrate (H 2 ) and product (H + ) pressure ( Fig. 2d ). We therefore titrated HydA1 to pH 4 before H 2 exposure, enhancing the proton pressure by four orders of magnitude ( Fig. 2c ). The presence of a band at 1,891 cm −1 in the resulting difference spectrum hinted at a minor contribution of H red , while no H sred could be detected. Instead, the H trans -like state represented the main fraction of our protein sample. No loss of cofactor was observed in the time frame of hours ( Supplementary Fig. 2a,b ), and the back-titration of HydA1 sample buffer from pH 4 to pH 8 clearly demonstrates a pH-dependent reversibility of the indicated state transitions ( Supplementary Fig. 2b,c ). The same applies for H 2 -dependency at pH 4 ( Supplementary Fig. 2d ). This bi-directionality is not compatible with the supposed H trans -like nature of the novel pattern [22] . Therefore, we will refer to this redox state in the following as H hyd . Similar results were obtained when repeating this experiment with samples of native DdH and CpI as representatives of the other two major [FeFe]-hydrogenase subtypes, implying this state and behaviour to be general features of the [FeFe]-hydrogenase family ( Supplementary Fig. 3 ). Figure 2: Population of H hyd in HydA1 by simultaneously increasing H 2 and H + pressure. ( a ) ATR FTIR difference spectrum (N 2 /pH8→H 2 /pH8), depicting the accumulation of the reduced states (H red /H red and H sred ) in the catalytic cycle of HydA1 under H 2 at pH 8. ( c ) ATR FTIR difference spectrum (N 2 /pH8→H 2 /pH4) depicting the accumulation of H hyd in the catalytic cycle of HydA1 under H 2 at pH 4. Catalytic cycles ( b , d ) beside the corresponding spectra illustrate the shift in steady-state equilibrium depending on applied substrate and product pressures in the working model of the catalytic cycle, which comprises the already-characterized states H ox , H red /H red and H sred , and the missing H 2 -activated state (H hyd ). Peak labels for H ox are presented in black, for H hyd in blue, for H red in green and for H sred in magenta (red asterisks: H red ). For the complete state-specific CN − -/CO-vibrational spectra of HydA1 observed during sample analysis, see Supplementary Table 1 . At pH 4, the vibrational signals of H ox were slightly shifted to higher frequencies (for more information see Supplementary Table 1 , Hox-blue). Full size image The influence of proton-transfer efficiency As the H 2 /H + balance appears to affect the electronic configuration of the H-cluster, alternative approaches were designed to enrich H hyd . HydA1 sample was once more purged with H 2 aerosol to first enrich the reduced states. When humidity was removed from the H 2 gas stream, sample films reacted by rapid dehydration. As predicted, this as well leads to a loss of H red /H sred in favour of the 1,978/1,960/1,860 cm −1 pattern ( Supplementary Fig. 4a ) indicating that the loss of bulk water has a similar effect to lowering the buffer pH, likely due to subsiding proton-transfer efficiency [24] ( Supplementary Fig. 4 ). To verify that an interference with the PTP enhances the population of the H hyd state under H 2 exposure, we blocked the PTP in HydA1 and CpI via site-directed mutagenesis at two strictly conserved positions for each protein. Position 1 (C169 of HydA1/C299 of CpI; Fig. 1 ), which was shown in earlier experimental data to be involved in catalytic proton transfer [3] , [5] , marks the most proximal position of the PTP to the 2Fe H sub-cluster, while position 2 (E141 of HydA1/E279 of CpI; Fig. 1 ) is situated more distant from the H-cluster. An exchange to alanine almost completely abolished H 2 -release activity for all variants ( Supplementary Fig. 6 ). To probe the structural integrity and unequivocally connect the monitored effects to an interrupted PTP, we solved the crystal structure of CpI E279A ( Fig. 3 ). The X-ray structure illustrates a fully intact H-cluster and overall identical structural features compared to wild-type CpI (refs 19 , 25 ), with the exception of the clearly diminished electron density at position 279, which is in full accordance with an exchange from glutamate to alanine. As a consequence of this non-conservative exchange, the path of polar side chains is interrupted between S319 and the harnessed H 2 O molecule. Figure 4a,b shows the reaction of enzyme variants C169A of HydA1 and E279A of CpI towards H 2 (black graph) at pH 8. 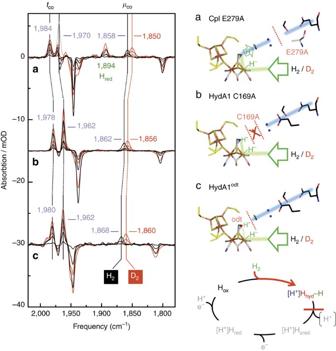Figure 4: Manipulating H+transfer traps the Hhydstate under H2or D2regardless of buffer pH. Left: ATR FTIR difference spectra (N2/pH8→H2or D2/pH8) depicting the accumulation of Hhydfor variants of the PTP E279A (CpI) (a) and C169A (HydA1) (b), as well as HydA1odt(c) under H2or D2at pH 8. The grey spectrum inadepicts the absolute absorption bands of Hhyd. Negative bands are assigned to Hox(Supplementary Table 1). Right: location of the corresponding PTP manipulation illustrated in a crystal structure model of CpI (pdb ID: 4XDC). Accumulation of Hhydunder D2(red spectra) does not affect the tCO-frequencies but induces a selective redshift for the μCO signal of 6–8 cm−1in all analysed variants. For the complete state-specific CN−/CO-vibrational spectra observed during sample analysis, seeSupplementary Table 1. 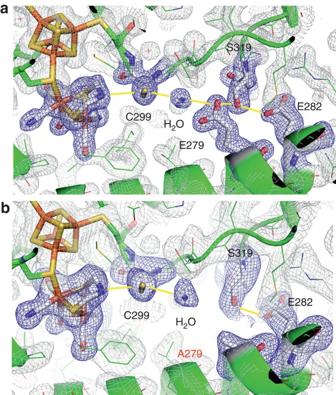Similar to the effect of acidification or sample drying, the oxidized state is lost in favour of bands at 1,978/1,962/1,863 cm −1 or 1,985/1,970/1,858 cm −1 , respectively. Figure 3: Crystal structure of the PTP in wild-type CpI and PTP-defective CpI variant E279A. Stick models and simulated annealing omit |Fo–Fc| electron density maps (blue) of the 2FeHcluster, and the amino-acid residues and the H2O molecules involved in proton transfer embedded in the 2Fo–Fc electron density maps (grey) of the X-ray structures of CpI wild-type25(a) and variant E279A (b). The presumed H+-transfer pathway is indicated in yellow. Crystal structure data for wild-type CpI correspond to pdb database entry 4XDC25. Details of the crystallographic data of E279A are summarized inSupplementary Table 2. For stereo view presentations seeSupplementary Fig. 9. Figure 3: Crystal structure of the PTP in wild-type CpI and PTP-defective CpI variant E279A. Stick models and simulated annealing omit |Fo–Fc| electron density maps (blue) of the 2Fe H cluster, and the amino-acid residues and the H 2 O molecules involved in proton transfer embedded in the 2Fo–Fc electron density maps (grey) of the X-ray structures of CpI wild-type [25] ( a ) and variant E279A ( b ). The presumed H + -transfer pathway is indicated in yellow. Crystal structure data for wild-type CpI correspond to pdb database entry 4XDC [25] . Details of the crystallographic data of E279A are summarized in Supplementary Table 2 . For stereo view presentations see Supplementary Fig. 9 . Full size image Figure 4: Manipulating H + transfer traps the H hyd state under H 2 or D 2 regardless of buffer pH. Left: ATR FTIR difference spectra (N 2 /pH8→H 2 or D 2 /pH8) depicting the accumulation of H hyd for variants of the PTP E279A (CpI) ( a ) and C169A (HydA1) ( b ), as well as HydA1 odt ( c ) under H 2 or D 2 at pH 8. The grey spectrum in a depicts the absolute absorption bands of H hyd . Negative bands are assigned to H ox ( Supplementary Table 1 ). Right: location of the corresponding PTP manipulation illustrated in a crystal structure model of CpI (pdb ID: 4XDC). Accumulation of H hyd under D 2 (red spectra) does not affect the tCO-frequencies but induces a selective redshift for the μCO signal of 6–8 cm −1 in all analysed variants. For the complete state-specific CN − /CO-vibrational spectra observed during sample analysis, see Supplementary Table 1 . Full size image We further exploited the effect of H hyd accumulation as a consequence of PTP obstruction to elucidate the proposed role of the azadithiolate ligand in the heterolytic cleavage of H 2 . The earlier-described procedure of in vitro maturation allows for the replacement of the native 2Fe H site with derivatives such as odt-2Fe H , which contains an oxodithiolate group ((SCH 2 ) 2 O,odt) instead of the native azadithiolate ((SCH 2 ) 2 NH, adt) [4] , [25] , [26] . After in vitro maturation with odt-2Fe H in presence of H 2 , HydA1 odt exhibits an infrared band pattern that strongly resembles H hyd (refs 23 , 26 ). The oxidized state of HydA1 odt was obtained via extensive purging with humidified N 2 . Subsequent exposure to H 2 induced a decrease in the H ox pattern in favour of bands 1,980, 1,962 and 1868, cm −1 ( Fig. 4c , black graph), however at a significantly lower rate compared to the corresponding experiment with wild-type HydA1. A terminal hydride in wild-type [FeFe]-hydrogenases To confirm the presence of a terminal hydride (t-H − ) in H hyd for wild-type hydrogenase and all examined variants, we probed the effect of an H/D isotope exchange on the FTIR band position of the bridging CO ligand, μCO (see Fig. 4 , red graph, and Supplementary Figs 7 and 8 including Supplementary Note 1 ). Terminal hydride species on metal carbonyl complexes are vibrationally coupled with the ligand positioned in trans due to resonant frequencies [27] . Previously published DFT calculations on the H-cluster model of HydA1 variant C169S predict a selective ‘redshift’ of 6 cm −1 for the μCO frequency as a consequence of substituting a hydride for a deuteride species located trans to μCO (ref. 23 ). When switching the purging gas from H 2 to D 2 , CpI E279A ( Fig. 4a ) and HydA1 C169A ( Fig. 4b ) showed a selective shift to lower energies by 5–6 cm −1 of the band at 1,860 cm −1 , which corresponds to the stretching vibration of μCO. A similar ‘redshift’ was observed for HydA1 odt when the oxidized enzyme was extensively treated with D 2 ( Fig. 4c and Supplementary Fig. 7b ). In Supplementary Fig. 8 we show spectra that document the H/D effect on wild-type HydA1 in presence of pH 4 and H 2 /D 2 . This confirms the corresponding behaviour of the H hyd state for all protein variants examined here. Le Chatelier’s principle was applied to enrich the highly transient H-cluster intermediate H hyd , which according to the current working model of catalytic H 2 turnover is predicted to carry a terminal hydride species. By simultaneously enhancing substrate and product pressure, we accumulated H hyd for three different wild-type [FeFe]-hydrogenases. Interestingly, a nearly identical FTIR band pattern was observed in our earlier spectroscopic analysis of the largely inactive HydA1 PTP variant C169S (ref. 28 ). Using DFT calculations, Mulder et al . [15] , [23] assigned this band pattern and redox species to a model of C169S that carried a terminal hydride at Fe d ( Supplementary Note 1 and Supplementary Fig. 5 ). Accumulation of H hyd was also observed on decreasing the humidity level of the protein sample. Recently, we demonstrated that freeze-drying renders [FeFe]-hydrogenase samples insensitive to O 2 exposure [24] . Although X-ray absorption spectroscopy data showed the formation of a stable O 2 adduct at the 2Fe H site, H-cluster degradation was not initiated, as opposed to hydrated enzyme in presence of O 2 (ref. 29 ). DFT calculations suggested a protonation step mandatory for generating destructive reactive oxygen species [30] . Therefore, a lack of H + -transfer activity in the freeze-dried state appeared to be a plausible explanation for this effect and dehydration should have a similar effect as lowering the pH. It can be speculated that the loss of bulk water, being the acceptor pool for exported protons, leads to an accumulation of protons in the PTP from the inside. Accordingly, low pH and dehydration both provide a counter pressure that prevents the H 2 -activated state from being deprotonated and proceeding to the reduced states ( Supplementary Fig. 4b,c ). The N 2 /H 2 difference spectra of site-directed exchange variants of HydA1 and CpI targeting positions C169/C299 and E141/E279 clearly demonstrate how the disrupted proton transport stabilizes the H hyd state regardless of buffer pH. This highlights that the transient character of H hyd essentially depends on a functional catalytic proton transfer, just as predicted from the working model ( Figs 1 and 2 ). In return, the analogous behaviour of cysteine and glutamate variants provides experimental proof for the involvement of the median glutamic acid residue (E141 HydA1 /E279 CpI ) in the proton-transfer mechanism of [FeFe]-hydrogenases. In future mutagenesis studies on the PTP of [FeFe]-hydrogenases, accumulation of H hyd can be regarded as an experimental indicator for the involvement of peptide positions in the catalytic H + transfer. The relevance of the bridgehead position of the 2Fe H subcluster for catalytic proton transfer was clearly demonstrated by the fact that cofactor variant HydA1 odt could be trapped in H hyd under H 2 independent of the pH, thus confirming the results of earlier studies, which pointed out the essential role of the native adt ligand as a proton relay to the substrate-binding site at Fe d . The fact that H 2 exposure of HydA1 odt results in H hyd accumulation suggests that the ether bridgehead of odt is capable to serve as a Lewis base and supports heterolytic H 2 cleavage. This reflects earlier investigations of Barton et al ., [31] which demonstrated in a comparative study, including different diiron complexes that the weakly basic ether group of odt can assist in proton relay during H 2 evolution [31] . However, in contrast to C169A and E279A, the H hyd spectrum of HydA1 odt could only be regained very slowly in presence of H 2 . While all examined enzyme variants exhibited an impaired proton transfer, for C169A and E279A the defect was restricted to the H + transfer across the protein shell ( Fig. 4 ). In case of HydA1 odt , the impairment already affected proton abstraction during H 2 heterolysis. This finding experimentally verifies the hypothesis that the pending amine group in the native adt ligand significantly enhances the rate of heterolytic H 2 cleavage [31] . The selective shift of the μCO band observed in H hyd on H/D exchange suggests the presence of a terminal hydride ligand for all PTP variants and catalytically competent wild-type enzymes examined here. In addition, two recently published studies independently demonstrated a terminal hydride for inactive HydA1 variants assigned to the presumptive H hyd state. Reijerse et al . [32] reported the direct detection of Fe d -H bending vibrations via nuclear resonance vibrational spectroscopy of a terminal hydride species in HydA1 odt after isolation under H 2 . This is in good agreement with our real-time analysis of HydA1 odt . Furthermore, Mulder et al . [15] applied electron paramagnetic resonance and Mössbauer spectroscopy to provide experimental support for the presence of a metal hydride species in HydA1 variant C169S, which largely adopted H hyd on supplementation with NaDT. Well in agreement with electrochemistry studies on HydA1 under turnover conditions [14] , the authors determined a H hyd transition potential close to the H 2 /H + redox couple. This argues in favour of the relevance of H hyd in the catalytic cycle. Both HydA1 C169S and HydA1 odt have been shown to be largely inactive [4] , [15] , [23] , [25] , [26] , [28] , [32] , and a definite proof for the catalytic relevance of H hyd can only be given by monitoring the succession of states during catalysis at sub-turnover time resolution as previously done for [NiFe]-hydrogenase [16] . However, this work strongly suggests that H hyd , as identified by Mössbauer and nuclear resonance vibrational spectroscopy, corresponds to the first transient state in the catalytic mechanism of H 2 oxidation and is shared by all major subtypes of [FeFe]-hydrogenases. It is therefore plausible to assume that we successfully accumulated a state carrying a terminal hydride ligand in native [FeFe]-hydrogenases. In response to modulating substrate and product concentrations (H + /H 2 ), accumulation of H hyd was found to be fully reversible showing that H hyd is no artificial dead-end state but part of the dynamic redox equilibrium typically occurring in the catalytically competent enzyme. All available data strongly suggest that H hyd is indeed the missing link in the catalytic mechanism of [FeFe]-hydrogenases. Site-directed mutagenesis of HydA1 and CpI Plasmids pET21b-HydA1Cr and pET21b-CpI were used as templates for site-directed mutagenesis, which was performed according to the QuikChange-PCR protocol published by Zheng et al . [33] For generating the constructs encoding HydA1 variants C169A, C169S and E141A, the 5′-overlapping mismatch primer pairs 5′-CAGCGCGTGTCCGGGCTGGATTGC-3′/5′-CCGGACACGCGCTGGTAAACATCGG-3′, 5′-CAGCTCATGTCCGGGCTGGATTGC-3′/5′-CCGGACATGAGCTGGTAAACATC-GG-3′ and 5′-CATCATGGAAGCGGGCAGCGAACTGCTGCATCGTC-3′/5′-GCAGTTC-GCTGCCCGCTTCCATGATGGTCAGATCC-3′ were used, respectively. For substitutions C299A and E279A within the polypeptide of CpI, primer pairs 5′-CCTCTGCGTGCCCAGGTTGGGTACGTC-3′/5′-CCTGGGCACGCAGAGGTAAACATT-GGGAAAGGG-3′ and 5′-CCAGTTCGGTAGCCGCTTCCATAATGGTCATATC-3′/5′-TG-GAAGCGGCTACCGAACTGGTTCAACG were utilized. Heterologous expression of HydA1 and CpI proteins The original plasmids pET21b-HydA1Cr and pET21b-CpI and their mutagenesis constructs were used for the heterologous expression of wild-type enzymes and variants of HydA1 and CpI (refs 4 , 25 , 34 , 35 ). Apo-forms of CpI and HydA1 (lacking 2Fe H ) were expressed anaerobically in Escherichia coli strain BL21 ΔiscR (ref. 36 ). Cells first grew aerobically in lysogeny broth (LB) medium pH 7.4 (0.1 M morpholineopropanesulfonic acid (Mops)-NaOH) supplemented with 5 g l −1 glucose and 2 mM ammonium iron citrate until an OD600 of 0.35–0.6 was reached. Before switching to anaerobic cultivation, the culture was flush with N 2 for 30 min to remove residual O 2 and supplemented with 25 mM sodium fumarate. Induction of gene expression was initiated by adding 5 mM cysteine and 0.5 mM β- D -1-thiogalactopyranoside. Cells were collected after 16–24 h expression via centrifugation. Purification of [FeFe]-hydrogenase apo-proteins The apo-proteins of wild-type and mutant forms of HydA1 and CpI, containing the 4Fe H subcluster but lacking the 2Fe H moiety, were expressed under anaerobic conditions in E. coli strain BL21 ΔiscR as described earlier [4] , [34] , [36] . After cell disruption via ultrasonication and the separation of the soluble proteins from the cell debris by ultracentrifugation and subsequent filtering (pore size 0.2 μm), we exploited the C-terminally fused Strep-tag-II sequence (WSHPQFEK) for protein purification, performing affinity chromatography with Strep-Tactin Superflow resin (IBA GmbH) in 100 mM Tris-HCl buffer (pH 8) supplemented with 2 mM NaDT. Protein purity was verified by SDS–PAGE and protein concentration determined via Bradford assay (BioRad). Synthesis of 2Fe H cofactor complexes The native-like 2Fe H -cofactor-mimic complex [Fe 2 [μ-(SCH 2 ) 2 NH](CN) 2 (CO) 4 ][Et 4 N] 2 (adt-2Fe H ) and its odt derivative [Fe 2 [μ-(SCH 2 ) 2 O](CN) 2 (CO) 4 ][Et 4 N] 2 (odt-2Fe H ) were synthesized according to literature procedures [25] . In vitro maturation To obtain the fully equipped holoprotein, heterologously expressed wild-type and mutant apo-proteins of HydA1 and CpI were maturated in vitro by adding adt-2Fe H (odt-2Fe H ) to a 10-fold excess in 0.1 M K 2 HPO 4 /KH 2 PO 4 buffer (pH 6.8), supplemented with 2 mM NaDT. To ensure complete sample maturation, the reaction mix was incubated for 1 h at room temperature. The resulting holoproteins were cleaned from surplus 2Fe H complex by size-exclusion chromatography using NAP 5 columns of GE Healthcare and concentrated in Amicon Ultra centrifugal filters 30K (Millipore). Afterwards, methyl viologen-specific H 2 production activity was determined to assess catalytic competence. In vitro assay to determine H 2 production activity H 2 production activities have been determined in vitro for wild-type and mutant proteins using 0.2 μg ml −1 of in vitro maturated [FeFe]-hydrogenase in 2 ml of 100 mM postassium phosphate buffer, pH 6.8, supplemented with 100 mM NaDT and 10 mM methyl viologen. Suba-seal vessels were sealed with stoppers, degassed for 5 min with 100% Argon and incubated for 20 min in a shaking water bath adjusted to 37 °C. For product quantification, 400 μl of sample head-space was analysed via gas chromatography (Shimadzu GC 2010). When enzyme activity was below the detection limit, the assay was repeated with a 10-fold increased enzyme concentration (2 μg ml −1 ). Crystallization and structure analysis of CpI variant E279A Using a 1:1 mix of E279A holoprotein (10 mg ml −1 ) and reservoir solution (0.1 M MES, pH 6, supplemented with 0.4 M MgCl 2 , 24% polyethylene glycol and 16% glycerol) in a hanging drop vapour diffusion set-up, single cuboid-shaped crystals of brownish colour were identified after 2–4 days at 277 K under anaerobic conditions. The selected protein crystal was mounted into a CryoLoop (Hampton Research) and flash-frozen in liquid N 2 . Diffraction data were collected at 100 K at beamline ID23-2 of the ESRF in Grenoble, France and processed using the software package XDS [37] . Molecular replacement and structure optimization were achieved with the software packages PHENIX [38] and Coot [39] . For details on crystallographic data of CpI E279A, see Supplementary Table 2 . Infrared spectroscopy All FTIR spectroscopy was conducted on a rapid-scan Tensor 27 spectrometer (Bruker Optik, Germany) equipped with a three-reflection ZnSe/silicon crystal ATR cell (Smith Detection, USA). The spectrometer was situated in an anaerobic gas chamber (Coy Laboratories, USA) in a water-free atmosphere of typically 99% N 2 and 1% H 2 . Supplementary Fig. 1 depicts the process flow diagram of the experimental set-up. Approximately 5 bar nitrogen carrier gas of ultra-high purity (5.0) was provided by a PN1450 nitrogen generator (Inmatec, Germany). The exact amount of N 2 was adjusted with a digital SmartTrak mass flow controller (MFC, Sierra, USA). Molecular H 2 (H 2 5.0, Linde, Germany) was injected separately via a second flow controller to create a well-defined mixture. The gas passed a 200 mbar check valve to protect the flow controllers from humidity. Afterwards, two sequential wash bottles (H 2 O and miscellaneous content, for example, buffer) could be switched into the gas stream. A bypass loop allowed for an adjustable proportion of the gas to bypass the wash bottles entirely or to run through the liquid volume to create a mix of carrier gas, water vapour and microscopic drops of liquid water (aerosol). The aerosol stream was fed to a customized polychlorotrifluoroethylene (PCTFE) gas cell, screwed gas-tight onto the ATR crystal plate. An exit line eventually guided the aerosol to a gas dump (fume). The PCTFE gas cell was equipped with three inlets and a manometer (not shown in Supplementary Fig. 1 ). Directly over the silicon crystal of the ATR unit, a cylindrical cavity joined all inlets. A gas-tight lid was screwed on top of the gas cell and allowed irradiation via an acrylic glass window. At this position, an infrared- or ultraviolet/visible-transparent window with protein sample could be adjusted into the aerosol stream. Thus, transmission samples for, for example, ultraviolet/visible or Raman spectroscopy could be prepared under the same conditions as monitored via the ATR silicon crystal. All spectra were recorded with 80 kHz scanning velocity, at a spectral resolution of 1 cm −1 , and varying extent of co-additions. All pH titrations were performed with citrate buffer (SSC). Data availability The atomic coordinates and factors for the reported crystal structure for CpI variant E279A have been deposited with the Protein Data Bank (PDB) under accession code 5LA3. Further data supporting the findings of this study are available within the article and its Supplementary Information file and from the corresponding authors on reasonable request. How to cite this article: Winkler, M. et al . Accumulating the hydride state in the catalytic cycle of [FeFe]-hydrogenases. Nat. Commun. 8, 16115 doi: 10.1038/ncomms16115 (2017). Publisher’s note : Springer Nature remains neutral with regard to jurisdictional claims in published maps and institutional affiliations.